Room temperature self-assembly of mixed nanoparticles into photonic structures Manufacturing complex composites and structures using incompatible materials is central to next-generation technologies. In photonics, silica offers passivity, low loss and robustness, making it the ideal material platform for optical transport. However, these properties partly stem from the high-temperature processing conditions necessary for silica waveguide fabrication, restricting the functionalisation of waveguides to robust inorganic dopants. This means for many sensor and active device applications, large numbers of materials are excluded. These include many organic and carbon systems such as dyes and diamond. Here we propose using intermolecular forces to bind nanoparticles together at room temperature and demonstrate the room-temperature self-assembly of long microwires (length ~7 cm, width ~10 μm) with and without rhodamine B. Further we report on mixed self-assembly of silica and single-photon-emitting nitrogen-vacancy-containing diamond nanoparticles, opening up a new direction in material science. There is a growing effort towards the integration of a wider range of materials onto key photonic platforms such as silicon [1] and silica [2] . Active functionalisation is often possible only through the integration of active materials [3] , [4] . For silica, the high temperatures used in manufacturing waveguides, unfortunately, makes it impossible to presently integrate a range of organic and inorganic species that are increasingly important for sensor and active waveguide devices. It is this fundamental disparity in processing regimes between different materials that poses a major research challenge in enabling new technologies. To address this problem, we focus on resolving the incompatibility issue of many organic and inorganic species in silica. In particular, we deal with a waveguide configuration that is attracting increasing current interest and relies on silica micro- and nanowires. The micro- and nanowire configuration is driven by a need for more compact and low-loss structures with high evanescent fields, useful in a broad range of applications spanning sensing [5] , lab-in-a-fibre, micro- and nano-photonics [6] through to optical interconnects for faster computing and signal processing with reduced thermal footprint computing [7] . This menagerie of applications illustrates how silica, along with silicon, remains one of the two key optical transport platforms in telecommunications and sensing. These photonic micro and nanowires are essentially waveguides with an air cladding, generating a high numerical aperture and permitting easy access to a significant evanescent field that is ideal for sensing and diagnostic applications, and for components. Across different material systems, numerous bottom-up approaches have been taken to manufacturing micro- and nanowires [8] , [9] , [10] , [11] using a variety of materials, such as silica, silicon, phosphate and various polymers [12] . For silica, the most successful approaches have been largely top–down tapering of optical fibres using CO 2 lasers [13] and naked flames [14] . Of these methods, nanowires drawn using a naked flame have produced the lowest transmission loss waveguides,<0.1 dB cm −1 . However, the problem with these methods is the need for high temperatures ( T >1,000 °C), which automatically prohibits the introduction of numerous organic and inorganic species. Many materials are increasingly being studied for use in photonics, electronics, photovoltaics and sensing, making their integration onto platforms, such as silica, important. These include conjugated and aromatic systems, diamond and other materials. Their integration into silica remains one of the great material challenges in chemistry, most commonly having relied on in-diffusion into porous silica structures such as sol–gel glass. So far, their integration into waveguides has also been restricted to post-manufacturing processes—one example is their incorporation into the air holes of structured optical fibres. Using this approach, the addition of porphyrins either by physisorption or chemisorptions has proved useful as acid sensors [15] . This approach is limited, however, by the need to post-include functionality that will adhere to the silica surface, and the loading of material is essentially restricted to monolayer thicknesses and is generally applicable only to compounds with intense light absorption. Another key material system attracting attention in photonics is diamond, especially nitrogen-vacancy (NV) centres within diamond nanoparticles. These are robust sources of photo-stable single photons at room temperature [16] , which also possess single-spin readout and quantum coherence [17] , making them a centrepiece of practical single-photon sources for quantum computing. Single-photon sources have been studied extensively since their discovery [18] and have been used for many applications [19] , [20] , [21] , [22] , including having been integrated within tellurite glass at a temperature of 700 °C and drawn into optical fibre [23] . The most significant attribute of single-photon emitters are that they can be used in quantum cryptography for secure communications and computing [24] . A manufacturing solution that allows fabrication of relatively low-loss photonic micro- and nanowires at cold temperatures with the dopants from the beginning will overcome these integration issues. Towards this end, we propose fabricating these wires in a novel bottom-up fabrication approach based on evaporative self-assembly of nanoparticles at room temperature combined with intermolecular attractive forces. This approach offers a new pathway for controlling and changing the composition of the waveguide (applicable more broadly to most material systems) for any desired application, as intermolecular forces, regardless of the identity of the species, are in most cases attractive. At room temperature, evaporation, ablation and other inhibitive processes normally present can all be circumvented by relying on van der Waals forces and lowest free-energy packing configurations alone. This approach makes it possible to include an array of chemical or nanoparticle species into silica microwires that would ordinarily be incompatible, overcoming the limitation of previous ‘hot’ methods and greatly expanding their possible uses in a range of different fields. To demonstrate this we focus on two examples of wide contemporary interest: one is the integration of low-temperature combustible, conjugated organic molecules into silica, and the second is the integration of diamond nanoparticles containing NV centres for single-photon emission. Intermolecular forces allow diverse particle mixing to fabricate new composite systems of materials that would not ordinarily be envisaged—in this case, a complex composite material involving silica and single-photon emitter containing diamond nanoparticles is demonstrated. This lays the foundation for a new approach, based on self-assembly, to enabling future quantum communications and optical computing, and more. We note that the technology of using intermolecular forces to circumvent the limits of more commonly used fabrication methods is not limited to silica and can be applied to any nanoparticle system. Self-assembly of silica nanoparticles The silica nanoparticles ( φ ~20 to 30 nm) are suspended in a polar solvent, H 2 O, with trace amounts of NH 4 + to overcome van der Waals attractive forces and prevent aggregation. Rhodamine B or nanodiamonds ( φ ~50 nm), were introduced into the silica dispersion and mixed thoroughly. Under ambient pressure and temperature ( T =295 K and P =1 atm), as the solvent is evaporating, the nanoparticles are able to aggregate [25] , assisted by convective flow within the drop, and through attractive intermolecular forces slowly pack into a crystal-like configuration of lowest energy. Consequently, the nanoparticle solution was deposited onto clean glass substrates to grow the microwires. As they dry, through surface and internal tensions, they may rise up detaching from the substrate. 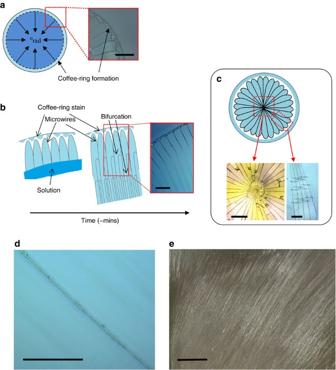Figure 1: Self-assembly and wire formation from a colloidal dispersion. (a) The schematic shows the formation of a ‘coffee-ring stain’ as the solvent starts to evaporate (the fine dashed line corresponds to initial solvent front, that is, the outer edge of the ring; the coarse dashed line corresponds to current solvent front, that is, the interior edge of the ring). The nanoparticles begin coalescing once the drop begins receding. Through van der Waals forces, the nanoparticles stick and attempt to pack into the lowest free-energy hexagonally close packed or body-centred cubic lattices. The optical image shows a section of such a drop where the coffee-ring effect is present. As the evaporating drop recedes towards the centre, radial compressive stresses inwards are established. (b) Here we illustrate how within a larger drop diameter (φ~20 cm), where the taper angle towards the centre is significantly less, the stresses involved with the nanoparticle packing can equal or exceed the radial stress so that secondary bifurcating fractures are formed, which propagate in parallel with each other, allowing long and uniform waveguides to form. (c) For small drop sizes this leads to fracturing towards the drop centre, forming tapers with an angle dependent on drop diameter. (d) An optical microscope image of a section of a typical microwire with widthw=6.81 μm at both ends of section of lengthl=0.5 mm. (e) Digital photograph of a batch of uniform, approximatelyl>5 cm long microwires fabricated on a glass substrate. All scale bars ina–dcorrespond to 200 μm; the scale bar inecorresponds to 1 cm. Figure 1a–c summarises the formation mechanism of the microwires relating to geometric stress and fracturing, which leads to uniform microwire formation—a more detailed description of the process is given in the Discussion. Typical silica microwires fabricated by this process are rectangular (cross-sectional area=24 μm 2 ) chosen to match the mode-field radius of standard telecommunications fibre, SMF-28, in cross-section. Lengths l ≥7 cm ( Supplementary Fig. s1a ) have been produced generating ultra-high aspect ratios ( l/w >7 × 10 3 ; Supplementary Fig. S1b shows a visual representation of microwire growth and dimension characterisations of microwires in a single drop). An optical microscope image of a silica microwire shows ( Fig. 1d ) a typical width of ( w =6.81 μm) and complete width uniformity within the section of length l =0.5 mm. A digital photograph ( Fig. 1e ) of an array of ultra-long ( l >5 cm) microwires, self-assembled from a single drop on a large glass substrate, shows the uniformity and reproducibility of the technique. 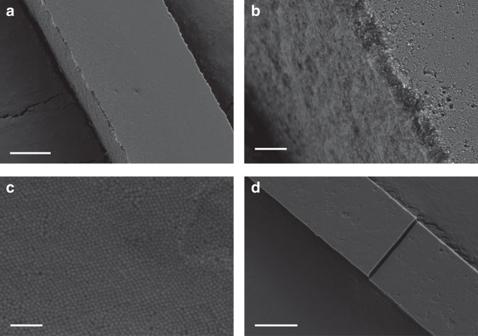Figure 2: Scanning electron microscope images of the silica microwires. (a) Typical self-assembled silica microwire with rectangular cross-sectional dimensions (25 × 10) μm. Scale bar corresponds to 10 μm. (b) Close-up of the same microwire showing smooth top surface and slightly rougher break (side) surface. Scale bar corresponds to 1 μm. (c) Extreme close-up of the smooth surface showing close packed structures. Scale bar corresponds to 200 nm. (d) A cleave induced by stress fracture manually applied using a ceramic tile—sharp cleaves are important when removing end-face scattering losses and integrating with other waveguide or optical fibre systems. Scale bar corresponds to 10 μm. Figure 2a shows a scanning electron microscope image of a microwire and its rectangular cross-section. Figure 2b are higher-magnification images revealing the hexagonally close packed and body-centred cubic lattice structure, which are the lowest free-energy configurations (almost the same) for the packing of uniform hard spheres ( η ~0.74%) [26] . The microwires are robust enough to be readily cleaved, similar to optical fibres, using a ceramic (Al 2 O 3 ) tile to introduce a stress fracture as shown in Fig. 2d . Figure 1: Self-assembly and wire formation from a colloidal dispersion. ( a ) The schematic shows the formation of a ‘coffee-ring stain’ as the solvent starts to evaporate (the fine dashed line corresponds to initial solvent front, that is, the outer edge of the ring; the coarse dashed line corresponds to current solvent front, that is, the interior edge of the ring). The nanoparticles begin coalescing once the drop begins receding. Through van der Waals forces, the nanoparticles stick and attempt to pack into the lowest free-energy hexagonally close packed or body-centred cubic lattices. The optical image shows a section of such a drop where the coffee-ring effect is present. As the evaporating drop recedes towards the centre, radial compressive stresses inwards are established. ( b ) Here we illustrate how within a larger drop diameter ( φ ~20 cm), where the taper angle towards the centre is significantly less, the stresses involved with the nanoparticle packing can equal or exceed the radial stress so that secondary bifurcating fractures are formed, which propagate in parallel with each other, allowing long and uniform waveguides to form. ( c ) For small drop sizes this leads to fracturing towards the drop centre, forming tapers with an angle dependent on drop diameter. ( d ) An optical microscope image of a section of a typical microwire with width w =6.81 μm at both ends of section of length l =0.5 mm. ( e ) Digital photograph of a batch of uniform, approximately l >5 cm long microwires fabricated on a glass substrate. All scale bars in a – d correspond to 200 μm; the scale bar in e corresponds to 1 cm. Full size image Figure 2: Scanning electron microscope images of the silica microwires. ( a ) Typical self-assembled silica microwire with rectangular cross-sectional dimensions (25 × 10) μm. Scale bar corresponds to 10 μm. ( b ) Close-up of the same microwire showing smooth top surface and slightly rougher break (side) surface. Scale bar corresponds to 1 μm. ( c ) Extreme close-up of the smooth surface showing close packed structures. Scale bar corresponds to 200 nm. ( d ) A cleave induced by stress fracture manually applied using a ceramic tile—sharp cleaves are important when removing end-face scattering losses and integrating with other waveguide or optical fibre systems. Scale bar corresponds to 10 μm. Full size image Optical characterisation of silica microwires Absorption and fluorescence measurements of the wires self-assembled from combined silica and rhodamine B solutions were obtained as shown in Fig. 3 (details in Methods). 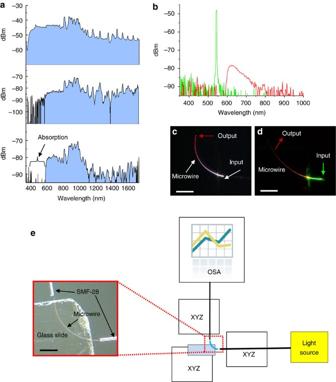Figure 3: Optical transmission and fluorescence measurements. (a) Top panel shows the transmission spectrum of the white light source through a normal SMF-28 fibre for reference; the middle panel shows the transmission spectrum of the white light source through an undoped silica microwire. The overall transmission loss is due to insertion losses made up, in part, by coupling loss and Rayleigh scattering from the silica nanoparticles. The bottom panel shows the transmission spectra of the white light source through a rhodamine B-doped microwire; transmission loss belowλ=590 nm compared with the undoped wire is due to optical absorption by the rhodamine B, which has an absorption band centred aboutλ=520 nm. (b) Fluorescence spectrum recorded using a HeNe laser (λ=543 nm) as the pump source. Transmission of 543 nm laser line is observed in the undoped microwire (green line), whereas the green light is absorbed by rhodamine B within the doped microwire (red line) and fluoresces in the red (λ~620 nm) as shown. (c) Optical image of the microwire used inato measure the absorption of rhodamine B. The microwire used has dimensionsw=30 μm,h=20 μm and radius of curvature ofRcurv=2.4 mm. White light was inserted into the microwire, and the red colouring at the output is due to absorption of green by the rhodamine B. (d) Optical image of the microwire used inbto measure the fluorescence of rhodamine B. The microwire has dimensionsw=30 μm,h=20 μm and radius of curvature ofRcurv=4.1 mm. A HeNe laser (λ=543 nm) was used as the pump source; the red colouring at the output of the microwire is due to rhodamine B fluorescence. (e) Schematic of the optical characterisation set-up: a rhodamine B-doped curved microwire (to prevent stray light from the input fibre reaching the collecting fibre) is supported on a glass slide. Two standard SMF-28 fibres were used to couple light into the microwire and to collect light at the output end, transmitting to an optical spectrum analyser (OSA). Three micropositioner (XYZ) stages are used to align the fibres and microwire. All scale bars correspond to 0.50 mm. Figure 3a shows the absorption of rhodamine B within the microwire as loss in signal power below λ =600 nm (bottom panel), and the white light profile and undoped microwire spectra (top and middle panel, respectively) are presented to contrast between the doped microwire. Figure 3b shows the fluorescence (red line) emission of the rhodamine B doped within the silica microwires when pumped with the green HeNe laser ( λ =543 nm); the green spectra shows the same pumping source through an undoped microwire where no fluorescence is observed. Figure 3c shows the coupling of white light through a curved microwire where the green absorption of the rhodamine B leads to a red colouring of the microwire towards the output end. Similarly, Fig. 3d shows coupling of the green HeNe laser ( λ =543 nm), which excites rhodamine B ( λ max =552 nm), generating strong fluorescence in the red. Figure 3e shows the experimental set-up of the light guidance measurements shown in Fig. 3a . The self-assembled silica microwire has a propagation loss of α =1.47 dB mm −1 (s.d., σ =0.78) for 10 measurements of microwires with dimensions of w =22 μm (s.d., σ =5) at λ =633 nm ( Supplementary Fig. S2 and Supplementary Methods ). The best-performing microwire has been measured with a loss of 0.46 dB mm -1 at λ =633 nm with dimension of ( w =23 μm) using the cut-back method. The total insertion loss of a doped microwire is estimated to be <30 dB above 600 nm from the transmission measurements ( Fig. 3a ) and arises principally from mode mismatch, coupling loss and attenuation on the glass slide. Figure 3: Optical transmission and fluorescence measurements. ( a ) Top panel shows the transmission spectrum of the white light source through a normal SMF-28 fibre for reference; the middle panel shows the transmission spectrum of the white light source through an undoped silica microwire. The overall transmission loss is due to insertion losses made up, in part, by coupling loss and Rayleigh scattering from the silica nanoparticles. The bottom panel shows the transmission spectra of the white light source through a rhodamine B-doped microwire; transmission loss below λ =590 nm compared with the undoped wire is due to optical absorption by the rhodamine B, which has an absorption band centred about λ =520 nm. ( b ) Fluorescence spectrum recorded using a HeNe laser ( λ =543 nm) as the pump source. Transmission of 543 nm laser line is observed in the undoped microwire (green line), whereas the green light is absorbed by rhodamine B within the doped microwire (red line) and fluoresces in the red ( λ ~620 nm) as shown. ( c ) Optical image of the microwire used in a to measure the absorption of rhodamine B. The microwire used has dimensions w =30 μm, h =20 μm and radius of curvature of R curv =2.4 mm. White light was inserted into the microwire, and the red colouring at the output is due to absorption of green by the rhodamine B. ( d ) Optical image of the microwire used in b to measure the fluorescence of rhodamine B. The microwire has dimensions w =30 μm, h =20 μm and radius of curvature of R curv =4.1 mm. A HeNe laser ( λ =543 nm) was used as the pump source; the red colouring at the output of the microwire is due to rhodamine B fluorescence. ( e ) Schematic of the optical characterisation set-up: a rhodamine B-doped curved microwire (to prevent stray light from the input fibre reaching the collecting fibre) is supported on a glass slide. Two standard SMF-28 fibres were used to couple light into the microwire and to collect light at the output end, transmitting to an optical spectrum analyser (OSA). Three micropositioner (XYZ) stages are used to align the fibres and microwire. All scale bars correspond to 0.50 mm. Full size image Single-photon emission from within a silica microwire The nanodiamonds containing single-NV point defect centres were sourced from a commercial supplier (NaBond). Typical particle sizes were φ ~50 nm, about double that of the silica nanoparticles. These were readily introduced into the water and dispersed amongst the silica particles. Despite the size difference, we successfully introduced these into the wires during self-assembly and characterised them using scanning confocal microscopy at room temperature. 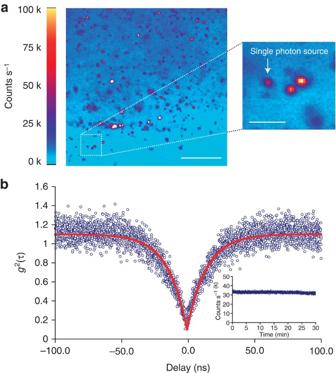Figure 4: Single-photon detection from nanodiamonds embedded in silica microwire. (a) A scanning confocal map of the photoluminescence from a nitrogen-vacancy (NV) defect centre with the nanodiamond is obtained over a (40 × 40)-μm2region of a nanodiamond-embedded silica microwire sample (image is taken from the top surface of the microwire; scale bar corresponds to 10 μm). The zoomed region shows NV photoluminescence intensity from an embedded single-photon emitter (scale bar corresponds to 2 μm). Counts shown were recorded from a single-photon detector. (b) Background corrected second-order autocorrelation function (blue circles) of a single-NV centre embedded in the silica microwire, shown ina, measured at room temperature. The value ofg2(0)~0.1 indicates single-photon emission. The solid red line represents a single exponential fit of the photon statistics. The inset shows the photostable emission from the single emitter identified ina. Figure 4a shows a 40 × 40 μm 2 region of a nanodiamond-embedded silica microwire sample, and the 5 × 5 μm 2 zoomed region shows NV-centre photoluminescence intensity from an embedded single-photon emitter. The photon statistics of the single-NV centre shown in the zoomed image in Fig. 4a were measured at room temperature (excitation: 0.5 mW at λ ex =532 nm) and the background corrected correlation function [27] , g 2 ( t ), is shown in Fig. 4b . The lowest measured value of g 2 (0) ~0.1 indicates that a single-photon emitter was addressed. The solid red line in Fig. 4b represents a single exponential fit of the photon statistics. The measured single-photon emission rate on one detector was ~30 k counts s −1 under the same excitation conditions, and the photostable emission collected for 30 min from the emitter can be observed in the insert of Fig. 4b . Figure 4: Single-photon detection from nanodiamonds embedded in silica microwire. ( a ) A scanning confocal map of the photoluminescence from a nitrogen-vacancy (NV) defect centre with the nanodiamond is obtained over a (40 × 40)-μm 2 region of a nanodiamond-embedded silica microwire sample (image is taken from the top surface of the microwire; scale bar corresponds to 10 μm). The zoomed region shows NV photoluminescence intensity from an embedded single-photon emitter (scale bar corresponds to 2 μm). Counts shown were recorded from a single-photon detector. ( b ) Background corrected second-order autocorrelation function (blue circles) of a single-NV centre embedded in the silica microwire, shown in a , measured at room temperature. The value of g 2 ( 0 )~0.1 indicates single-photon emission. The solid red line represents a single exponential fit of the photon statistics. The inset shows the photostable emission from the single emitter identified in a . Full size image The formation of microwires is due to several geometric-related stresses invoked by the close packing of the silica nanoparticles as the solvent evaporates and the volume recedes. The initial stress build-up within the drop structure is the radial stress, pointing inwards to the centre of the drop as the drop recedes; this initially leads to formation of a so-called ‘coffee-stain ring’ [28] ( Fig. 1a ). The wire formation preferentially occurs in the direction of the evaporating solvent front; in combination with aggregation and packing, the one-dimensional recession drives the formation of rectangular, or slab, waveguides. The attractive van der Waals forces and close packing of the nanoparticles in effect attempts to resist these compressive stresses. As the self-assembly propagates following the evaporation front, radial compressive stresses continue to build up until uniform and periodic fracturing ( σ radial > σ fract(thres) ) occurs around the perimeter of an ideally round coffee stain. In the case of small volumes, the radial component is not overcome by resisting packing forces, and tapered structures are created ( Fig. 1c ). For larger drops, where the radial component has a smaller angle from the natural plane of cleaving along the mostly bcc-like packing of the nanoparticles, stresses again build up but are less and can be overcome by packing stresses that also build up. This time a secondary, parallel bifurcating fracture occurs, and this is the point at which it is possible to generate uniform waveguides ( Fig. 1b ). By controlling the drop size and concentration of nanoparticles in water, tens to hundreds of microwires up to a few centimeters in length have been produced from a single drop ( Fig. 1e ) demonstrating that, in principle, a low-cost mass production is possible. The cross-sectional dimensions also vary depending on concentration, and the lower the nanoparticle concentration the longer and thinner the wires ( Supplementary Fig. S3 ). By varying all these parameters, microwires with cross-sectional widths between 2 and 150 μm were fabricated, with no obvious restriction to this range if further improvements are aimed for. This flexible window allows for mode matching to a range of optical fibres and waveguides. The microwires are mechanically robust, easily handled and manipulated onto a customised optical waveguide characterisation set-up as well as mounted for optical and scanning electron microscope imaging. The silica microwires reported here have relatively low propagation loss ( α =1.47 dB mm −1 ) compared with other optical microwire. Mitsui et al . [11] have reported formation of colloidal wires via a templating method using polystyrene spheres with losses of α ~2.0 dB per 10 μm, and Barrelet et al . [7] have reported losses of α ~1.0 dB per 10 μm in CdS nanowires. Tong et el . [14] have reported losses of <0.1 dB cm −1 at λ =633 and 1,550 nm for their tapered silica microwire, which is single mode with adiabatic input and output coupling. In these experiments, our self-assembled silica microwires are multimode with V >~132 ( V =((2 πw )/ π ) NA ), assuming a rotationally invariant analogue microwire with width w =30 μm carrying λ =1,550 nm light. Multimode operation of the microwire was also confirmed by mode imaging in the far-field as shown in Supplementary Fig. S4 , where we observe the complex interference pattern arising from the various modes supported on the microwire. For optical sensing work, multimode propagation is often used as a means of increasing the collection angle of a fibre or waveguide, and therefore the signal-to-noise ratio, compared with single-mode waveguides. An estimate of the refractive index of the silica microwire is n ~1.475, similar to that of individual silica nanoparticles as expected and reported by Khlebtsov et al . [29] This value is slightly higher than fused silica ( n =1.458) and quartz ( n =1.458), reflecting the tight packing of the nanoparticles. Although the losses of the individual silica microwires cannot be directly compared because of the different preparation and measurement techniques, the microwire reported here is the first self-assembled silica wire. Its total insertion loss, α <30 dB, is a level well above what can be achieved with improved waveguide matching and coupling. It lies between that of the top–down fabricated silica optical fibre tapers and that of other templated colloidal microwires made from other semiconductor materials. We believe the insertion losses should be able to approach the best adiabatic tapers produced by top–down, high-temperature drawing, as there is no intrinsic material loss, and this is the subject of further work. In conclusion, the self-assembled silica microwires, doped with rhodamine B and self-assembled with nanodiamonds, reported here have the potential for a host of optical interconnect, sensing, laser, optical diagnostic and quantum applications. The silica nanoparticle platform (or any other nanoparticle platform) combined with our cold fabrication process allows total integration of new materials into existing silica communications and sensor networks, as well as in many other application areas such as photovoltaics, biodiagnostics and so on. It opens up a vast field for compositional control of other organic and inorganic chemicals within silica waveguides (or any other nanoparticle platform) for applications in opto-electronics (for example, graphite), photovoltaics (for example, customised porphyrins and metals), plasmonics and metamaterials (for example, metals) and novel optical circuitry (for example, magnetic materials). We have also introduced, using silica nanoparticle and diamond nanoparticles twice the size, the concept of mixed nanoparticle self-assembly of composite structures and new materials based on intermolecular forces. Mixed self-assemblies will have unique, perhaps entirely novel, packing topologies dependent on relative attractive forces and different sizes, laying a foundation for advanced material condensation studies with molecular parallels. Further, there is no reason why the process could not be adapted to grow directly onto existing technologies including, for example, wires (or self-assembled films, and other micro and nano structures, possibly with exotic dopants) attached to silicon waveguides. Self-assembly of silica microwires The microwires were self-assembled from individual silica nanoparticles with diameters between φ ~20 to 30 nm in an aqueous colloidal dispersion (5% w/w, pH=9 with NH 4 + counterions) onto glass substrates. The glass substrate was first cleaned by methanol and then the silica dispersion (volume depends on length required: for l= 7 cm long wire, V= 4 ml was used) was deposited on top using a hand-held pipette with a nozzle diameter of 2 mm. The solvent was left to evaporate at ambient pressure and temperature (1 atm, 295 K). Integration of rhodamine B and nanodiamonds Both the organic fluorescent marker—rhodamine B ([9-(2-carboxyphenyl)-6-diethylamino-3-xanthenylidene]diethylammonium chloride (C 28 H 31 ClN 2 O 3 ); m =0. 1 mg) and the nanodiamonds ( m =0.1 mg), were introduced in solid form to different silica dispersions (5% w/w, H 2 O; V =2 ml). The mixture was then stirred for 10 min, followed by utlrasonication for a further 10 min to allow dissolution. The glass slide was first wetted by methanol ( V =100 μl) and then the silica dispersion ( V =100 μl) was deposited on top using a hand-held pipette with a nozzle diameter of 2 mm. The solvent was left to evaporate at ambient pressure and temperature (1 atm, 295 K). Optical characterisation of self-assembled silica microwires The propagation of light within the silica microwire waveguides was characterised using several different sources, including red and green HeNe lasers ( λ =633, 543 nm) and a white light source (1,000 W Xe lamp). Input and output lights were delivered by a standard SMF-28 telecommunication optical fibre, whereas transmission spectra were collected on an optical spectrum analyser. Sources of transmission loss involved both mismatch between the current photonic microwire and the SMF-28 fibres, as well as attenuation from contact with the slide, with refractive index ( n =1.510). To obtain absorption and transmission measurements of rhodamine B absorption within the microwire, a butt-coupling set-up with three-axes micro-positioners was used. A curved silica microwire was placed on the edge of a low-index borosilicate glass slide, and two SMF-28 fibres guided light into the microwire and collected the light from the output, which was then processed on the optical spectrum analyser. The 90° curve ensured no stay light launched from the input fibre reached the collection fibre. An optical image of the set-up is shown in Fig. 3e . Imaging and single-photon correlation measurements A custom-built scanning confocal microscope, with a × 100 (numerical aperture=0.95) air objective and bandpass filter ( λ em =650–750 nm), was used to measure the NV-centre emission from the silica–nanodiamond samples. Photon statistics from each fluorescent region on the confocal images were studied using a Hanbury Brown and Twiss interferometer [30] to identify single-NV centres. The photon statistics were measured at room temperature with a laser excitation power of 0.5 mW at λ ex =532 nm. The background corrected correlation function, g 2 ( t ), was determined using the methods described in [27] , and is shown in Fig. 4b ; the single emitter was found to exhibit a characteristic single-photon dip in the second-order correlation function, g 2 (0), at 0 delay time ( t =0). How to cite this article: Naqshbandi, M. et al . Room temperature self-assembly of mixed nanoparticles into photonic structures. Nat. Commun. 3:1188 doi: 10.1038/ncomms2182 (2012).